The B-type response regulator GmRR11d mediates systemic inhibition of symbiotic nodulation Key to the success of legumes is the ability to form and maintain optimal symbiotic nodules that enable them to balance the trade-off between symbiosis and plant growth. Cytokinin is essential for homeostatic regulation of nodulation, but the mechanism remains incompletely understood. Here, we show that a B-type response regulator GmRR11d mediates systemic inhibition of nodulation. GmRR11d is induced by rhizobia and low level cytokinin, and GmRR11d can suppress the transcriptional activity of GmNSP1 on GmNIN1a to inhibit soybean nodulation. GmRR11d positively regulates cytokinin response and its binding on the GmNIN1a promoter is enhanced by cytokinin. Intriguingly, rhizobial induction of GmRR11d and its function are dependent upon GmNARK that is a CLV1-like receptor kinase and inhibits nodule number in shoots. Thus, GmRR11d governs a transcriptional program associated with nodulation attenuation and cytokinin response activation essential for systemic regulation of nodulation. Symbiotic nodulation is imperative for the survival and productivity of legumes under nitrogen-limiting conditions. It is initiated upon plant perception of lipochitooligosaccharide Nod factors (NFs) released by rhizobia [1] , [2] and requires the coordination of rhizobial infection and root nodule organogenesis. The LysM-type receptor kinases (e.g., NFR1 and NFR5 in Lotus ( L .) japonicus , NFP in Medicago ( M .) truncatula and GmNFR1α and GmNFR5α in soybean) [3] , [4] , [5] , [6] , [7] , [8] , [9] recognize NFs and activate the NF signaling pathway involving the encoding/decoding of nuclear Ca 2+ oscillations, heteropolymerization of NODULATION SIGNALING PATHWAY 1 (NSP1)-NSP2 and activation of nodulation genes, such as NODULE INCEPTION ( NIN ) [10] , [11] , [12] . Nodule initiation largely depends on the locally produced phytohormone cytokinin (CKs) to allow root cortical cells to successfully dedifferentiate and proliferate in the initial stages of nodulation [13] , [14] , [15] , [16] , [17] . The levels of CKs in plants are regulated by the biosynthesis and metabolism of CKs. Here, the most prevalent active CK is trans -zeatin ( tZ ) and its biosynthesis is regulated by Isopentenyl transferases (IPTs) and the cytochrome P450 enzymes CYP735A1/2 [18] , [19] . The free base in active forms of CKs is catalyzed by LONGLY GUY (LOG) family enzymes CK nucleoside 5′-monophosphate phosphoribohydrolases [20] , [21] . CK levels are also modulated by sugar conjugation or via irreversible cleavage by cytokinin oxidases (CKXs) [22] . The biosynthesis and metabolism of CKs are dynamically regulated by endogenous developmental cues as well as abiotic and biotic stimuli [18] , [22] . In legumes, the expression of multiple CK synthesis genes is rapidly induced by rhizobia and NFs, resulting in an early burst of CKs [23] , [24] . Mutations in CK synthesis genes, such as ISOPENTENYL TRANSFRASE 3 ( IPT3 ) and IPT4 as well as several LOG genes ( LOG1/2/4 ) result in reduced nodulation [25] , [26] , [27] , [28] . Analogously, loss of function of the CYTOKININ OXIDASE/DEHYDROGENASE 3 ( LjCKX3 ) gene, which causes elevated root CK levels, also reduces the number of nodules [24] . Thus, the CK bioactive pool is precisely regulated during nodulation to maintain an optimal number of nodules in the root system. Plants perceive CKs via CK sensors histidine kinases (HKs) and transmit the signals to type-B response regulators (RRs) through authentic histidine phosphotransferase (AHPs), which then propagate the signaling by activating primary CK-responsive genes, including type-A RR genes [29] . The type-B RRs contain a receiver domain and a C-terminal extension including a Myb-like DNA binding domain. These type-B genes are not transcriptionally regulated by CKs, but they can directly bind to the specific motifs in the promoters of many CK-responsive genes in a CK-dependent manner to activate or repress these genes [29] , [30] . Thus, the type-B RRs are essential for the initial response to CKs at transcriptional level and can interact with transcription factors, such as TGA3 in salicylic acid (SA) and DELLA proteins in gibberellin (GA), to mediate the cross talks between CK and these hormonal signaling pathways [31] , [32] . Rhizobia inoculation can induce CK sensor genes, such as MEDICAGO CYTOKININ RESPONSE 1 ( MtCRE1 ) and LOTUS HISTIDINE KINASE 1 ( LHK1 ), to activate the CK signaling that is essential for nodulation [23] , [29] , [33] , [34] , [35] . Genetic mutations that impair CK perception and response can lead to altered nodulation. For example, gain-of-function mutations in MtCRE1 and LjLHK1 induce spontaneous nodules in the absence of rhizobia [33] , [35] , while loss-of-function mutations in MtRRB3 lead to the reduction of the nodulation [36] . Genetic data suggest that CKs act downstream of the CALCIUM-AND CALMODULIN-DEPENDENT PROTEIN KINASE (CCaMK) but upstream of NIN in the NF signaling pathway [33] . Notably, CKs induce the expression of NIN [16] , which conversely activates MtCRE1 [37] . CK-induced MtNIN also activates the symbiosis-specific gene MEDICAGO C-TERMINALLY ENCODED PEPTIDE 7 ( MtCEP7 ) to systemically positively regulate nodulation through its receptor, LRR-RLK COMPACT ROOT ARCHITECTURE 2 (MtCRA2), in shoots [38] . Therefore, CK and NF signaling pathways may converge at NIN to control root cellular fate and subsequent nodule formation. Symbiotic nodulation is achieved at the expense of legume growth. Plants have evolved an intrinsic control mechanism, called autoregulation of nodulation (AON), to systemically regulate nodulation so that plants can balance the carbon costs of growth and nodulation. During nodule formation, CK-induced NINs can directly activate the CLAVATA3/EMBRYO (CLE) coding genes MtCLE12/13 , lotus CLE-ROOT SIGNAL 1/2/3 ( LjCLE-RS1/2/3 ), and soybean RHIZOBIA-INDUCED CLE 1/2 ( GmRIC1/2 ) [39] , [40] , [41] . These peptide hormones are transported to the shoot to bind to their receptors, such as SUPER NUMERARY NODULE (SUNN), HYPERNODULATION AND ABERRANT ROOT 1 (HAR1), and Glycine max NODULE AUTOREGULATION RECEPTOR KINASE (GmNARK), which negatively regulate nodulation using long distance signals [42] , [43] , [44] , [45] . The CKs synthesized in shoots have been proposed to function as mobile signals to inhibit nodulation by suppressing NIN [26] , [46] . It has long been proposed that shoot-controlled nodulation acts downstream of CK signaling-mediated activation of nodule initiation [33] . Additionally, Lotus uses an LHK1-dependent feedback mechanism from the root cortex to the epidermis, which is coupled to AON to monitor and maintain rhizobial infection and nodule development [47] . Thus, CKs may trigger the onset of both local and systemic negative feedback loops through NIN. Given the important role of CKs in nodulation homeostasis, there has been increased interest in CK-mediated local and systemic regulation of nodulation. However, the mechanisms that modulate CKs to elicit an optimal response of legumes to rhizobia are not fully understood. In this work, we identified a B-type RR transcription factor GmRR11d as an important effector of AON that represses GmNIN1a expression. We showed that GmRR11d expression is responsive to both CKs and rhizobia, but oppositely regulates plant response to CKs and nodulation in soybean. GmRR11d can directly bind to the promoter of GmNIN1a to repress its transcription, and CKs can enhance the binding of GmRR11d to GmNIN1a promoter. In addition, we found that GmRR11d interacts with GmNSP1a, which is an upstream transcriptional activator of GmNIN1a , to suppress its transcriptional activity on GmNIN1a expression. We also demonstrated that GmRR11d functions downstream of GmNARK to control root nodulation. Collectively, our findings elucidate a molecular mechanism that regulates nodulation homeostasis by elevating the CK sensitivity of infected root and by attenuating CK-activated nodulation via a systemic negative feedback loop. Identification of GmRR11d as a GmNSP1-interacting protein As NSP1 activates the expression of NIN , which is an evolutionarily conserved and coordinating regulator of CK-mediated nodulation and nodulation autoregulation in legumes [46] , [48] , we hypothesized that AON might induce a transcription factor that suppresses the transcriptional activity of NSP1, resulting in repression of NIN and attenuation of nodulation. To test this hypothesis, we first examined the expression of two soybean NSP1 ortholog genes ( GmNSP1a and GmNSP1b ) and evaluated the effect of individual loss-of-function mutations in GmNSP1a and GmNSP1b on nodulation of soybean. GmNSP1a and GmNSP1b were differentially expressed during rhizobial infection and nodule development. GmNSP1a was induced by rhizobia rapidly and remained at higher expression levels during nodulation. GmNSP1b was initially downregulated after rhizobial inoculation; it was then upregulated during rhizobial early infection and peaks when nodule formed, and then gradually decreasing during nodule development (Supplementary Fig. 1a, b ). Gene knockout using CRISPR/Cas9 and phenotypic analysis showed that loss of function mutations in GmNSP1a and GmNSP1b resulted in reduced numbers of nodules, suggesting that both GmNSP1a and GmNSP1b positively regulate nodulation in soybean (Supplementary Fig. 1c–g ; Supplementary Fig. 2 ). Next, we performed a yeast-two-hybrid (Y2H) screen in a soybean nodulation cDNA library using GmNSP1a as a bait to identify the GmNSP1a-interacting proteins. Interestingly, a RR protein (Glyma.18G010800) was identified as a putative GmNSP1a-interacting protein. This protein is the soybean homolog of Arabidopsis RR11 (ARR11) (Supplementary Fig. 3 ), a B-type RR protein [49] . Genome-wide analyses identified four copies of ARR11 genes ( Glyma.11G246400 , Glyma.05G144500 , Glyma.08G100900 and Glyma.18G010800 ) in soybean, which were named GmRR11a, GmRR11b, GmRR11c and GmRR11d based on their protein homology to ARR11 (Supplementary Fig. 3 ). These GmRR11s contain conserved receiver domains (REC) and MYB (DNA-binding domain) domains, similar to their putative orthologs in M. truncatula , L. japonicus and A. thaliana (Supplementary Fig. 4a ). The putative GmNSP1a-interacting protein GmRR11d is the shortest one compared to GmRR11a/b/c, with significant sequence variations in its C-terminal amino acids compared with ARR11 (Supplementary Fig. 4b ). To validate the interaction between GmRR11d and GmNSP1a, we performed Y2H, bimolecular fluorescence complementation (BiFC), co-immunoprecipitation (CoIP), pull-down and localized surface plasmon resonance (LSPR) assays. The interaction between GmRR11d and GmNSP1a was detected in both S. cerevisiae cells and in the nucleus of N. benthamiana leaf cells (Supplementary Fig. 5 and Fig. 1a ), which is consistent with the nuclear localization of GmRR11d and GmNSP1a (Supplementary Fig. 6 ). The in vivo interaction between GmRR11d and GmNSP1a was confirmed by CoIP (Fig. 1b ). The in vitro direct interaction between GmRR11d and GmNSP1a was verified by pull-down and LSPR assays (Fig. 1c and Supplementary Fig. 7 ). NSP1 promotes nodulation by forming a co-transcriptional activator complex with NSP2 [48] . There are two soybean NSP2 ortholog genes (named GmNSP2a and GmNSP2b ) (Supplementary Fig. 8 ). Both GmNSP2 genes showed a similar pattern of induction by rhizobia and are required for nodulation of soybean (Supplementary Fig. 9 ). To test whether the GmRR11d-GmNSP1a interaction is specific, we analyzed whether GmRR11d could interact with GmNSP2 using GmNSP2a as an example. GmNSP2a was present in the nucleus (Supplementary Fig. 6 ), which is different from the reticulum/nuclear envelope localization of MtNSP2 before NF treatment [12] . It appeared that GmRR11d did not interact with GmNSP2a in either the Y2H, CoIP or the pull-down assays, but it did interact with GmNSP2a in N. benthamiana leaf cells and LSPR assay (Fig. 1a, c and Supplementary Fig. 5 and Supplementary Fig. 7 ). These results suggest that GmRR11d, a B-type RR protein, may be involved in GmNSP1a-regulated nodulation pathway. Fig. 1: GmRR11d interacts preferentially with GmNSP1a. a BiFC assay to detect the interactions between GmRR11d and GmNSP1a or GmNSP2a. The interactions between GmRR11d and GmNIN1a [41] , GmNSP1a or GmNSP2a, and STF1 [83] were used as negative controls. Four independent experiments were repeated with similar results. Scale bars = 100 μm. b CoIP assay of interaction between GmRR11d and GmNSP1a. GmRR11d-6xMYC (58 kDa) alone or GmRR11d-6xMYC and GmNSP1a-3xHA (63 kDa) were transiently expressed under the control of the 35 S promoter in N. benthamiana leaves. GmRR11d-6xMYC immunoprecipitated from total protein extracts. Three independent experiments were repeated with similar results. c Pull-down assays to show that MBP -GmRR11d (91 kDa) interacts with GST-GmNSP1a (87 kDa) but not GST-GmNSP2a (82 kDa). Three independent experiments were repeated with similar results. Full size image GmRR11d positively regulates root sensitivity to cytokinin ARR11 plays an important role in the CK-induced root growth response in Arabidopsis [49] . To explore whether GmRR11d mediates the root response to cytokinin 6-Benzylaminopurine (BAP) in soybean, we expressed GmRR11d driven by the CaMV35S (35 S) promoter in the wild-type (Wm82), and the empty vector (EV) was used as a control. qRT-PCR analysis showed that GmRR11d expression was significantly induced by low concentration of BAP (0.001 μM) but returned to the basal level in high concentration of BAP in roots expressing empty vector (EV1); the transgenic roots expressing 35 S:GmRR11d exhibited markedly elevated expression of GmRR11d compared with the vector control roots regardless of BAP concentration (Fig. 2a ). Intriguingly, the transgenic roots overexpressing GmRR11d exhibited enhanced sensitivity to cytokinin-induced growth inhibition compared to the vector control (Fig. 2b, c ). To validate the role of GmRR11d in CK response of soybean, we also analyzed the CK sensitivity of the RNAi-GmRR11d hairy roots. As expected, RNAi-GmRR11d transgenic roots exhibited substantially reduced cytokinin sensitivity (Fig. 2d–f ). These results indicate that GmRR11d acts as a positive regulator of CK signaling and the plant CK response in soybean. Fig. 2: GmRR11d is CK responsive and positively regulates the sensitivity of soybean roots to CKs. a Relative expression of GmRR11d in transgenic roots expressing 35 S : GmRR11d treated with BAP of different concentrations (0, 0.001, 0.1, 1 μM). The expression levels were normalized against the geometric mean of soybean GmELF1b . Data are presented as means ± SD from three biological replicates. Different letters indicate significant differences at p < 0.05 (Two-way ANOVA). b Length of hairy roots expressing EV1 and 35 S : GmRR11d treated with different concentrations (0, 0.001, 0.1, 1 μM) of BAP for 6 days ( n ≥ 6). Data are presented as means ± SE. Different letters indicate significant differences at p < 0.05 (Two-way ANOVA). c Representative images of individual root overexpressing GmRR11d and the EV1. Three independent experiments were repeated with similar results. Scale bars = 1 cm. d Relative expression of GmRR11d in transgenic roots expressing RNAi - GmRR11d treated with BAP of different concentrations (0, 0.001, 0.1, 1 μM). The expression levels were normalized against the geometric mean of soybean GmELF1b . Data are presented as means ± SD from three biological replicates. Different letters indicate significant differences at p < 0.05 (Two-way ANOVA). e Length of hairy roots expressing EV2 and RNAi - GmRR11d treated with different concentrations (0, 0.001, 0.1, 1 μM) of BAP for 6 days ( n ≥ 6). Data are presented as means ± SE. Different letters indicate significant differences at p < 0.05 (Two-way ANOVA). f Representative images of individual root downregulating GmRR11d and the EV2. Three independent experiments were repeated with similar results. Scale bars = 1 cm. Full size image To confirm the effect of GmRR11d on the plant response to cytokinin, we analyzed the expression levels of GmRR15a and GmRR15b , the closest homologs of Arabidopsis ARR7 and ARR15 (Supplementary Fig. 10 ), which are CK-inducible type-A ARR genes in Arabidopsis [50] . Indeed, both GmRR15a and GmRR15b were induced by exogenous CKs (Supplementary Fig. 11a ). In the GmRR11d -overexpressing hairy roots, the transcript levels of both genes were significantly higher than that in the vector control roots following cytokinin treatments, especially the level of GmRR15b (Supplementary Fig. 11b, c ), suggesting that the cytokinin hypersensitive phenotype of GmRR11d -overexpressing roots is mainly due to elevated expression of these cytokinin-responsive genes. Together, these results suggest that GmRR11d is a typical type-B transcription factor and regulates the transcriptional and physiological responses of soybean roots to CKs. GmRR11d is induced by rhizobia and is highly expressed in nodules To investigate whether GmRR11d is involved in nodulation, we first analyzed the expression of GmRR11d . Results from qRT-PCR analyses showed that GmRR11d was expressed at the highest level in mature nodules compared with in leaves and roots at 28 days after inoculation (DAI) (Fig. 3a ). Further gene expression analysis revealed that GmRR11d was rapidly induced by rhizobia in soybean roots, peaked at 3 DAI and returned to its original level at 6 DAI (Fig. 3b ). GmRR11d expression was then gradually increased and reached its second peak when nodule became mature at 21 DAI (Fig. 3b ). To further understand the cellular expression pattern of GmRR11d , we generated a construct expressing the GUS gene under the control of the 2-kb promoter of GmRR11d . Histochemical analysis of GmRR11d expression showed that GmRR11d was induced by rhizobia and expressed throughout the whole nodule formation process (Fig. 3c–p ). GmRR11d was highly expressed in nodule primordia (Fig. 3k) , in basal emerging and young nodules (Fig. 3l, m ) and in intact mature nodules (Fig. 3n ). Cross-sectional analysis showed that GmRR11d was mainly expressed in the cortex of the young and mature nodules (Fig. 3o, p ). These results suggest a probable role of GmRR11d in nodule organogenesis in soybean. Fig. 3: The expression pattern of GmRR11d during nodulation. a , b qRT-PCR analysis of GmRR11d expression in different tissues or during nodulation stages. a Roots, leaves, and nodules of soybean seedlings inoculated with B. diaefficiens strain USDA110 were harvested at 28 DAI and used for gene expression analyses. GmELF1b was used as the endogenous control gene. Data are presented as means ± SD from three biological replicates. More than 6 samples were analyzed in each independent biological repeat. Different letters indicate significant differences at p < 0.05 (One-way ANOVA). b Seven-day-old seedlings were inoculated with B. diaefficiens strain USDA110 and the infected root materials were collected at 0, 1, 3, 6, 12 HAI and 1, 3, 6,10, 14, 21, 28 DAI for expression analysis of GmRR11d . GmELF1b was used as the endogenous control gene. The data are shown as the means ± SD from three biological replicates. Asterisks indicate significant differences relative to 0 HAI (Two-sided Student’s t -test, * p < 0.05; ** p < 0.01; *** p < 0.001). c – p Histochemical assay of proGmRR11d : GUS and in the transgenic roots and nodules. Three independent experiments were repeated with similar results. c – j Representative GUS staining in hairy roots of proGmRR11d : GUS . GUS activity was monitored at 12 HAI c , d , 1 DAI e , f , 3 DAI g , h and 6 DAI i , j with B. diazoefficiens USDA110. Scale bars = 100 μm in c – j . k – n The expression pattern of GmRR11d in emerging nodule k , young nodule l and mature nodule m , n . o , p Cross-sectional analysis of the expression pattern of GmRR11d in young and mature nodules, the red arrows show cortex. Scale bars = 1 mm in k – p . Full size image GmRR11d functions as a negative regulator in soybean nodulation To functionally validate the role of GmRR11d in nodulation, we generated hairy roots overexpressing GmRR11d ( 35 S : GmRR11d ) and evaluated the effect of 35 S : GmRR11d on nodule number at 21 DAI. Unexpectedly, the 35 S : GmRR11d roots produced significantly fewer nodules than the control roots by approximately 41% (Fig. 4a–c ), suggesting a negative regulatory role of GmRR11d in root nodulation of soybean. To investigate whether endogenous GmRR11d is a negative regulator of root nodulation, we then generated RNAi - GmRR11d composite plants to specifically knockdown the expression of GmRR11d (Fig. 4d and Supplementary Fig. 12 ). We found that GmRR11d knockdown significantly increased nodule numbers at 21 DAI and the number of root nodules per hairy root was almost doubled (Fig. 4e, f ). We also evaluated nodule number of GmRR11d knockout roots using CRISPR/Cas9 technology, and the result showed that loss of function mutations in GmRR11d caused significantly increased number of nodules (Supplemental Fig. 13a–e ). These results confirm that GmRR11d is a key negative regulator of soybean nodulation. Fig. 4: Alterations of GmRR11d expression affect nodulation. a – c Overexpression of GmRR11d reduces nodule number. a qRT-PCR analysis of transgenic hairy roots expressing 35 S : GmRR11d . The expression levels were normalized against the geometric mean of soybean GmELF1b . Data are presented as means ± SD from three biological replicates. Asterisks indicate significant differences relative to the EV1 control. Two-sided Student’s t -test *** p 0.001. b , c Quantification and representative images of nodule number per hairy root expressing EV1 and 35 S : GmRR11d . Data are presented as means ± SD (14 hairy roots in EV1 and 18 hairy roots in 35 S : GmRR11d ). Three independent experiments were repeated with similar results. Asterisks indicate significant differences relative to the EV1 control. Two-sided Student’s t -test, *** p < 0.001. Scale bars = 1 cm. d – f Knockdown of GmRR11d increases nodule number. d qRT-PCR analysis of transgenic hairy roots expressing RNAi-GmRR11d . The expression levels were normalized against the geometric mean of soybean GmELF1b . Data are presented as means ± SD from three biological replicates. Asterisks indicate significant differences relative to the EV2 control. Two-sided Student’s t -test, * p < 0.05. e , f Nodulation phenotypic analysis of individual hairy roots expressing EV2 and RNAi-GmRR11d at 21 DAI. Scale bars = 1 cm. Data are presented as means ± SD (24 hairy roots in EV2 and 28 hairy roots in RNAi-GmRR11d ). Three independent experiments were repeated with similar results. Asterisks indicate significant differences relative to the EV2 control. Two-sided Student’s t -test, *** p < 0.001. Boxes indicate the first and third quartiles and the whiskers indicate the minimum and maximum values, the black lines within the boxes indicate the median values and black circles mark the individual measurements. The numbers above the boxes in ( b ) and ( e ) represent the mean values. Full size image GmRR11d directly targets and represses the expression of GmNIN1a The facts that GmRR11d interacts with GmNSP1a and negatively regulates nodulation suggest that GmRR11d may inhibit nodulation by repressing the expression of GmNIN1a and its downstream genes. To prove this hypothesis, we examined the expression of GmNIN1a and the downstream marker gene GmENOD40-1 in 35 S : GmRR11d and RNAi - GmRR11d hairy roots at 2 DAI. Indeed, the expression of both GmNIN1a and GmENOD40-1 genes was significantly decreased in 35 S : GmRR11d transgenic roots while increased in RNAi - GmRR11d transgenic roots (Fig. 5a ). To further verify the negative regulatory effect of GmRR11d on GmNIN1a transcription, we transiently co-expressed proGmNIN1a : GUS with empty vector (EV1) or 35 S : GmRR11d in leaf epidermal cells of N. benthamiana leaves. The GUS assay showed that the expression of GmNIN1a was markedly decreased when proGmNIN1a : GUS was co-expressed with 35 S : GmRR11d (Fig. 5b, c ). The same result was observed when proGmNIN1a : GUS was co-expressed with 35 S : GmRR11d in the transgenic hairy roots of soybean compared with the empty vector (Fig. 5d ), suggesting that GmRR11d is indeed a transcriptional repressor of GmNIN1a . Fig. 5: GmRR11d directly targets the promoter of GmNIN1a and represses GmNIN1a expression. a qRT-PCR analysis of GmNIN1a and GmENOD40-1 expression in rhizobia-infected hairy roots expressing 35 S:GmRR11d or RNAi-GmRR11d at 2 DAI. The expression levels were normalized against the geometric mean of soybean GmELF1b . Data are presented as means ± SD from three biological replicates. More than 12 roots were analyzed in three independent biological repeats. Asterisks indicate significant differences relative to the EV1 or EV2 control. Two-sided Student’s t -test, * p < 0.05; ** p < 0.005. b – d GUS assays showing the specific binding of GmRR11d to the GmNIN1a promoter and the inhibitory effect of GmRR11d on GmNIN1a in N. benthamiana leaf ( b , c ; Scale bars = 1 cm) and in transgenic soybean hairy root ( d ; Scale bars = 100 μm). The proGmNIN1a and proGmNIN1a - DM contain normal (GGATT) and mutated (AAAAA) GmRR11d binding sites in GmNIN1a promoter, respectively. The construct harboring proGmNIN1a:GUS or proGmNIN1a-DM was co-transformed with empty vector (EV1) or 35 S:GmRR11d into epidermal cells of N. benthamiana leaves and transgenic hairy roots of soybean, and GUS staining were performed 48 h after transformation in N. benthamiana leaves and 2 DAI in transgenic hairy roots. Data are presented as means ± SD from three biological replicates. Different letters indicate significant differences at p < 0.05 (one-way ANOVA). e Diagram of the GmNIN1a promoters. GmRR11d binding site (GGATT) shown as purple boxes. The fragments marked by the letters A to G indicate the regions examined in ChIP-qPCR assays. Region A contains two GmRR11d binding sites. f ChIP-qPCR assay showing binding of GmRR11d to the GmNIN1a promoter. DNA fragments were co-immunoprecipitated with anti-FLAG antibody from chromatin suspensions prepared from 35 S : GmRR11d-FLAG or empty vector (EV1) samples. DNA fragments corresponding to the regions indicated in e were analyzed by qRT-PCR. The DNA fragments were normalized to the input data. Data are presented as mean ± SD of three biological repeats. Asterisks indicate significant differences relative to the EV1 control. Two-sided Student’s t -test, ** p < 0.01. Full size image Type-B RR transcription factors can directly bind and transactivate target genes [49] , [50] . Next, we analyzed a 3 kb promoter sequence of GmNIN1a and found that there are 7 B-type RR binding sites and 2 putative ARR11 binding sites (Supplementary Fig. 14a ), indicating that GmRR11d may directly bind to the GmNIN1a promoter and repress its expression. To test this hypothesis, we first conducted chromatin immunoprecipitation (ChIP) assays in soybean hairy roots at 6 DAI. We found that GmRR11d was significantly enriched at the promoter region containing two B-type RR binding sites GGATT of GmNIN1a (Fig. 5e, f and Supplemental Fig. 14a ). To validate the direct binding of GmRR11d to the specific region of the GmNIN1a promoter, we next performed a protein-DNA pull-down assay. For this experiment, we expressed and purified the full-length GmRR11d protein fused to maltose-binding protein (MBP), MBP-GmRR11d, in Escherichia coli . Indeed, MBP-GmRR11d was able to interact with DNA fragment containing GGATT (Supplementary Fig. 15 ). To confirm that GmRR11d represses GmNIN1a expression through the specific binding to the B-type RR binding sites in the promoter of GmNIN1a , we tested the binding activity of GmRR11d on the fragment containing the mutated GmRR11d binding site (AAAAA, mprobe) and the transcriptional activity of GmRR11d on the GmNIN1a promoter containing the mutated GmRR11d binding sites ( proGmNIN1a-DM ). The binding ability of GmRR11d on the mutated fragment was completely inhibited (Supplementary Fig. 15 ), as a consequence the transcriptional GmNIN1a repression by GmRR11d was completely blocked when proGmNIN1a-DM : GUS was co-expressed with 35 S:GmRR11d in N. benthamiana leaves and in hairy roots (Fig. 5b–d ). These results suggest that GmRR11d repression of GmNIN1a transcription plays a crucial role in the regulation of GmNIN1a and symbiotic nodulation in soybean. In addition to GmNIN1a , three additional orthologous NIN genes ( GmNIN1b , GmNIN2a , and GmNIN2b ) can be found in the soybean genome, which are also induced by rhizobia and mediate nodulation [51] . We then analyzed the expression levels of these GmNINs in 35 S : GmRR11d or Cas9-GmRR11d hairy roots. All tested genes displayed a similar expression pattern to GmNIN1a , with all genes showing increased expression levels in GmRR11d knockout roots while reduced expression levels in GmRR11d overexpression roots (Supplemental Fig. 13f, g ). These results indicate that GmRR11d may repress the expression of all these GmNIN genes. To prove this possibility, we analyzed the promoter sequences of the other three GmNIN genes and found many B-type RR binding sites in GmNIN1b, GmNIN2a and GmNIN2b promoter sequences (Supplemental Fig. 14a ). Further ChIP-qPCR assays verified that GmRR11d can bind to the B-type RR binding sites on the promoters of these three GmNINs (Supplemental Fig. 14b ). Taken together, these results demonstrate that GmRR11d can bind to and repress the expression of all the GmNIN genes during nodulation. GmRR11d inhibits the transcriptional activity of GmNSP1a The fact that GmRR11d and GmNSP1a antagonistically regulate GmNIN1a transcription prompted us to investigate the underlying molecular mechanism. To this end, we first performed protein domain mapping experiments to determine how GmRR11d and GmNSP1a interact using Y2H assays. Interestingly, we found that the C-terminus (CT) of both GmRR11d and GmNSP1a was sufficient for their interaction in S. cerevisiae (Supplementary Fig. 16 , Fig. 6a, b ). Notably, the C-terminus of GmRR11d has no conserved domain, while the C-terminus of NSP1a is a highly conserved GRAS domain consisting of five motifs, including LHRI, VHIID, LHRII, PFYRE, and SAW that are essential for its interaction with NSP2 and among them, the LHR1 and LHR2 motifs are responsible for the DNA binding activity of NSP1 [48] . To confirm which domain of the GmNSP1a C-terminus binds to GmRR11d, we further truncated the GRAS domain into LHR1, VHIID, LHR2, PFYRE, and SAW motifs and tested their interactions with GmRR11d. The result showed that all motifs except SAW interacted with GmRR11d (Fig. 6a, b ). The interaction between GmRR11d and GmNSP1a likely disrupts the ability of GmNSP1a to form a complex with GmNSP2 and its ability to bind to the DNA, such as binding to the GmNIN1a promoter. Fig. 6: GmRR11d interacts with GmNSP1a and inhibits its transcriptional activity. a Domain structure of GmNSP1a. b Domain mapping for the interactions between GmNSP1a or its derivatives and GmRR11d by Y2H assay. Three independent experiments were performed with similar results. c ChIP assay showing binding of GmNSP1a to GmNIN1a promoter and the inhibition effect of GmRR11d to the binding of GmNSP1a to GmNIN1a promoter. DNA fragments were co-immunoprecipitated with anti-GFP antibody from chromatin suspensions prepared from 35 S : GmNSP1a-GFP , 35 S : GmRR11d-GmNSP1a-GFP or control (empty vector) samples. DNA fragments corresponding to the regions indicated in Fig. 5e . Data are presented as means ± SD of three biological repeats. Different letters indicate significant differences at P < 0.05 (One-way ANOVA). d The expression level of GmRR11d and GmNSP1a in hairy root expressing 35 S : GmNSP1a-GFP or 35 S : GmRR11d-GmNSP1a-GFP . Data are presented as means ± SD of three biological repeats. More than 30 hairy roots were analyzed in three independent biological repeats. Different letters indicate significant differences at P < 0.05 (One-way ANOVA). e GUS activity of proGmNIN1a : GUS and proGmNIN1a-DM : GUS with different combinations with 35 S : GmRR11d , 35 S : GmNSP1a and 35 S : GmRR11d + 35 S : GmNSP1a in N. benthamiana leaves. Data are presented as means ± SD from three biological repeats. Different letters indicate significant differences at P < 0.05 (One-way ANOVA). Full size image To verify the effect of GmRR11d on the DNA binding of GmNSP1a, we conducted ChIP and EMSA assays. The ChIP assay confirmed that GmNSP1a was enriched in regions B and C of the GmNIN1a promoter, while the enrichment of GmNSP1a on GmNIN1a promoter was significantly reduced in the presence of GmRR11d (Fig. 6c, d ). Furthermore, our EMSA results also confirmed that the binding of GmNSP1a to the GmNIN1a promoter was negatively correlated with GmRR11d (Supplementary Fig. 17 ). Moreover, we performed GUS assays to validate the inhibitory role of GmRR11d on GmNSP1a activation of GmNIN1a transcription in vivo. GUS activity analysis showed that GmNSP1a can activate both wild type and the mutated ( proGmNIN1a-DM ) GmNIN1a promoters, but this activation was effectively suppressed by GmRR11d in N. benthamiana leaf cells (Fig. 6e , Supplemental Fig. 18 ). These results confirm the negative role of GmRR11d on GmNSP1a transcriptional activity and suggest that the binding of GmRR11d on GmNIN1a promoter is not essential for the inhibition of GmNSP1a-activated GmNIN1a expression. Thus, we conclude that GmRR11d interaction with GmNSP1a is sufficient to interrupt the binding of GmNSP1a to the GmNIN1a promoter. GmRR11d functions downstream of GmNARK to regulate nodule number Our results that GmRR11d was induced by rhizobia and reached its highest expression level at the onset of nodule formation but negatively regulated nodule number led us to hypothesize that GmRR11d may be upregulated by AON to inhibit further nodule formation. To test this hypothesis, we first assessed the effects of GmNARK on the transcription levels of GmRR11d . GmRR11d was induced by rhizobia and gradually increased as nodule development in roots of the wild-type ( Glycine max ) cv. Bragg (Fig. 7a, b ), which is similar to the pattern in Williams 82. In contrast, transcriptional induction of GmRR11d in the infected roots was almost completely blocked in the knockout mutant of GmNARK (supernodulating nitrate-tolerant symbiotic 1007 , nts1007 ) (Fig. 7a, b ). The results suggest that rhizobial induction of GmRR11d is likely to be dependent on the function of GmNARK. Fig. 7: GmRR11d acts as a downstream regulator of GmNARK in soybean. a , b The expression of GmRR11d in roots a and nodules b of wide-type cv Bragg and GmNARK mutant nts1007 . Seven-day-old-plants were inoculated with USDA110. The roots were harvested at 0, 1, 3, 5, and 10 DAI and the nodules were harvested at 6, 8, 10, 12, 14, 16, 18, and 25 DAI. Data are presented as means ± SD from three biological repeats. More than 9 samples were analyzed in three independent biological repeats. Asterisks indicate significant differences relative to the wild type control. Two-sided Student’s t -test, * p < 0.05; p ** < 0.01; *** p < 0.001. c The expression of GmRR11d in shoots and roots of Bragg/Bragg, Bragg/ nts1007 , nts1007 / nts1007 and nts1007 /Bragg grafting plants. Data are presented as means ± SD from three biological repeats and 6 samples were collected for expression analysis. Different letters indicate significant differences at P < 0.05 (One-way ANOVA). d The expression of GmRR11d in split-roots of Bragg and nts1007 . -R/-R and +R/ + R treatment as negative and positive control. Data are presented as means ± SD from three biological repeats and 12 roots were collected for expression analysis. Different letters indicate significant differences at p < 0.05 (Two-way ANOVA) e qRT-PCR analysis of GmRR11d in empty vector (EV1) and 35 S : GmRR11d transgenic hairy roots of Bragg and nts1007 plants. Data are presented as means ± SD from three biological repeats and more than 10 roots were collected for expression analysis Asterisks indicate significant differences relative to the EV1 control. Two-sided Student’s t -test, ** p < 0.01. f Nodule number of Bragg and nts1007 plants expressing EV1 and 35 S : GmRR11d at 21 DAI. Data are presented as means ± SD from three biological repeats and more than 10hairy roots were collected for analysis. Different letters indicate significant differences at p < 0.05 (Two-way ANOVA). g Phenotypes of nodules from individual hairy roots of Bragg and nts1007 plants expressing EV1 and 35 S : GmRR11d at 21 DAI. h BAP treatment increases the enrichment of GmRR11d in the promoter of GmNIN1a . DNA fragments were co-immunoprecipitated with anti-FLAG antibodies from chromatin suspensions prepared from 35 S:GmRR11d-FLAG or control (EV1) samples treated with or without 10 −7 M BAP. The DNA fragments were normalized to the input data. Data are presented as means ± SD from three biological repeats. Different letters indicate significant differences at p < 0.05 (one-way ANOVA). i A proposed working model for GmRR11d-mediated nodulation inhibition. At low nitrogen conditions, rhizobia infection induces GmNSP1a to activate GmNIN1a that promotes nodulation and autoregulation of nodulation (AON). At the early infection stage, the level of GmRR11d is low and CK level is suitable for nodulation, GmNSP1s complexes with GmNSP2 to activate GmNIN expression; activation of AON induces expression of B-type regulator GmRR11d which interacts with GmNSP1a and suppresses its transcriptional activation of GmNIN1a . Meanwhile, AON-induced CK accumulation enhances binding of GmRR11d to the GmNIN1a promoter to repress its expression induced by CK and to activate CK signaling, thereby inhibiting nodulation of soybean. Full size image To confirm that the failure of GmRR11d induction in nts1007 is caused by the function of GmNARK in shoots, we analyzed the expression of GmRR11d in grafted plants. Indeed, the level of GmRR11d expression was reduced when the plants were grafted with nts1007 mutant scions (Fig. 7c ). We further tested the expression of GmRR11d in a split-root system of the cultivar Bragg and nts1007 . qRT-PCR and GUS activity assays showed that GmRR11d expression was induced significantly in non-inoculated part compared with control in Bragg, but the induction of GmRR11d was blocked completely in nts1007 (Fig. 7d , Supplemental Fig. 19 ). These results demonstrate that GmNARK in shoots plays a key role in GmRR11d induction during nodulation. To determine the genetic relationship between GmNARK and GmRR11d , we overexpressed GmRR11d in wild-type Bragg and nts1007 mutant roots and evaluated the nodule number of the composite transgenic plants. qRT-PCR showed that the expression level of GmRR11d was substantially elevated in the transgenic hairy roots of both the wild type and nts1007 (Fig. 7e ). Overexpression of GmRR11d significantly reduced the number of root nodules in the wild type (Fig. 7f, g ), which is consistent with the results in Williams 82 (Fig. 4 ). The nts1007 mutant indeed exhibited a supernodulating phenotype, but interestingly, the number of nodules per transgenic hairy root of nts1007 overexpressing GmRR11d was dramatically decreased, and the supernodulating phenotype of the nts1007 mutant was almost completely rescued (Fig. 7f, g ). These results indicate that GmNARK may inhibit nodulation in shoots by inducing GmRR11d expression in roots. To further strengthen the relationship between GmRR11d and AON, we analyzed GmRR11d expression in the hairy roots overexpressing GmRIC1 and GmRIC2 . As expected, GmRR11d was upregulated in the hairy roots overexpressing GmRIC1 and GmRIC2 (Supplementary Fig. 20 ), supporting the notion that GmRR11d acts downstream of AON. Unexpectedly, the expression levels of GmRIC1 and GmRIC2 was upregulated in hairy roots overexpressing GmRR11d and downregulated in hairy root knockout GmRR11d (Supplementary Fig. 21 ), suggesting that GmRR11d also regulates AON through positive feedback. TOO MUCH LOVE ( TML ), which encodes a F-box protein and acts downstream of HAR1 is required for nodulation inhibition in L. japonicus [52] . To explore the possible relationship between GmRR11d and GmTML1b, a downstream negative regulator of AON, we measured the transcription level of GmRR11d in the hairy roots overexpressing GmTML1b and found that the level of GmRR11d expression remained unchanged (Supplementary Fig. 20 ). Furthermore, we found that GmTML1b expression was not altered in GmRR11d knockout roots compared with the vector control roots, although it was slightly upregulated in the hairy roots overexpressing GmRR11d (Supplementary Fig. 21 ). These results suggest that GmRR11d is a key component in the AON signalling but inhibits nodulation in a mainly GmTML1b-independent manner. Cytokinin promotes the binding of GmRR11d to the GmNIN1a promoter It has been shown that the transcription levels of B-type RR genes are not responsive to CKs, but the binding of type-B RR proteins to its target genes can be enhanced by CKs in Arabidopsis [30] . Unlike the Arabidopsis B-type RR genes, GmRR11d was induced by various concentrations of CKs (Fig. 2a ), we next wondered whether CKs can also enhance GmRR11d binding to the GmNIN1a promoter. To answer the question, we expressed 35 S:GmRR11d-FLAG in hairy roots of soybean in the absence or presence of CKs and performed a ChIP assay. The analysis result revealed that CK treatment promoted GmRR11d binding to the promoter region of GmNIN1a . In the absence of exogenous CKs, there was a low level of enrichment of GmRR11d at the binding site on the GmNIN1a promoter, but in the presence of CK treatment, there was a substantial increase in enrichment of GmRR11d on the GmNIN1a promoter region (Fig. 7h ). This result indicates that cytokinin can enhance GmRR11d binding to the GmNIN1a promoter. Maintaining the optimal nodule number in legumes requires coordination of nodulation and autoregulation of nodulation. When legume plants detect low nitrogen levels, they attempt to form root nodules by activating NIN through CKs [34] , [37] , [53] . Subsequently, activation of the AON pathway can alleviate CK-activated nodulation by suppressing NIN expression in roots [26] , [46] . Thus, the regulation of the CK-NIN axis is essential for the best outcomes in the trade-off between plant growth and symbiotic nodulation. Here, we found that the CK signaling type-B transcription factor GmRR11d is induced by rhizobia through AON signaling. GmRR11d is induced by CKs and upregulation of GmRR11d causes CK hypersensitivity of plants. We also found that GmRR11d negatively regulates nodulation by repressing transcription of GmNIN1a which is enhanced by CK, and by suppressing transcriptional activation activity of GmNSP1a on GmNIN1a . Our work reveals a novel mechanism that AON signaling maintains nodulation homeostasis through simultaneous induction of CK hypersensitivity and attenuation of GmNIN1a-mediated NF signaling during nodulation. Induction of transient CK biosynthesis and accumulation in the root susceptible zone is essential for nodule initiation [23] , [33] . However, excessive CK accumulation or exogenous CK treatments inhibits root nodulation [24] , [54] . In Lotus japonicus , AON signaling can induce overproduction of CKs in the shoot that transports to the infected root to suppress nodulation [26] , [33] . In addition, it has been shown that shoot control of root nodulation is at downstream of CK signaling-mediated activation of nodule initiation [33] , [47] . It is apparent that the regulation of the levels of CKs and/or CK response is central for nodulation homeostasis. It is likely that the NF and AON signaling pathways converge on, and dynamically regulate the levels and sensitivity of cellular CKs to control nodulation homeostasis in legumes. In this work, we provide evidences that AON can induce a type-B RR transcription factor in infected root that connects the AON, NF and CK signaling pathways to inhibit nodulation. Our results showed that a type-B RR transcription factor encoding gene GmRR11d is induced by rhizobia in soybean roots at the time when the AON signaling is switched on and its expression induction is largely dependent on the shoot GmNARK. In addition, GmRR11d expression is regulated by GmRIC1 and GmRIC2. Importantly, GmRR11d negatively regulates soybean nodulation in a GmNARK-dependent manner. Thus, GmRR11d is a key downstream component of the long-distance negative feedback loop during nodulation. It has been shown that TML targeted by miR2111 is a central factor at the downstream of AON in L. japonicus [52] , [55] . However, our data showed that GmRR11d and GmTML1b may suppress nodulation independently of each other in soybean. It is likely that GmRR11d and GmTMLs achieve the same out-put through different mechanisms in soybean. In L. japonicus and soybean, NIN activates the expression of CLE-RS1/RS2 and GmRIC1/GmRIC2 to turn on AON, which in turn leads to reduced expression of NIN and nodulation inhibition [41] , [46] . Decreased expression of NIN should lead to downregulation of CLE-RS1/RS2 and GmRIC1/GmRIC2 , thus attenuating AON as well. However, we found that although GmRR11d represses GmNIN1a expression, the expression of GmRIC1 and GmRIC2 in 35 S:GmRR11d roots increased rather than decreased. This is conceivable because AON is a continuous process that must occur during nodule formation and development. Given that GmRR11d and GmRIC1/2 genes have overlapping expression pattern in infection and nodule development [56] and there are GmRR11d binding sites in the promoters of GmRIC1 / 2 (Supplementary Fig. 22 ), it is likely that GmRR11d can directly activate the expression of GmRIC1 / 2 in a spatio-temporal manner. The fact that B-type RR transcription factors can regulate expression of a wide range of genes [30] , [57] supports our hypothesis. Further analyses of direct binding and activation of GmRR11d on GmRIC1 and GmRIC2 promoter would prove our hypothesis. Nodulation and nodulation inhibition are complex processes involving various hormones and multiple signaling pathways. Recently, GA was shown to activate AON through activation of NIN , suggesting more regulatory pathways that induce CLE-RS2 and GmRIC1/2 expression and activate AON [58] . B-type RRs can target various genes including the genes in hormone synthesis, metabolism and signal transduction [57] . Interestingly, all three important genes GmRR11d , GmRIC1, and GmRIC2 in AON are induced by CKs, suggesting a crucial role of CKs in autoregulation of nodulation, but we don’t exclude the possibility that GmRR11d activates GmRIC1 and GmRIC2 through other mechanisms. Based on these findings, we proposed that nodulation autoregulation is continuously activated and dynamically modulated during nodule development to maintain nodulation homeostasis although AON is activated early with nodule formation. Type-B RRs are indispensable for CK signal transduction and increasing the expression level of the genes results in hypersensitivity to CKs and altered growth and development in Arabidopsis [29] . Our results demonstrate that GmRR11d is a functional type-B RR transcription factor. It contains both receiver and Myb-like domains that are also found in other type-B RR proteins, and has DNA binding activity, and is localized in the nucleus. Our results also proved that GmRR11d mediates the activation of CK signal transduction as the increasing level of GmRR11d increases the sensitivity of soybean roots to CKs through induction of type-A RR genes, such as GmRR15a and GmRR15b . It is worthy to note that unlike other type-B ARRs in Arabidopsis (e.g., ARR10) [30] , the GmRR11d promoter contains RR DNA-binding sites and the expression of GmRR11d is induced by CKs; but like the type-B ARRs in Arabidopsis [30] , GmRR11d binding to its target DNA is also enhanced by low-level CKs. The results suggest that GmRR11d uses a conserved mechanism for mediating CK response of soybean. The induction of GmRR11d expression and increased DNA binding activity by CKs may result in greater transcriptional activity of GmRR11d in the regulation of CK responsive genes, such as GmRR15s and CK hyposensitivity that affects cell division and expansion [30] . Together with observations that AON induces GmRR11d expression in rhizobial infection and in nodule formation to inhibit nodulation, it is conceivable that AON signaling may also activate GmRR11d to induce CK hypersensitivity of infected root and developing nodule, thereby inhibiting nodulation. It remains unknown whether AON also induces biosynthesis of active CKs when AON is turned on, leading to induction and activation of GmRR11d to cause CK hypersensitivity and nodulation inhibition. It would be interesting to know whether and how AON activates GmRR11d , as well as GmRIC1 and GmRIC2 , to exert their inhibitory role during nodule organogenesis and development. Upon NFs perception, the NIN genes are essential for NF signal transduction. The spatial and temporal expression of NIN s and their levels are central for nodulation [10] , [37] , [41] , [46] , [59] , [60] . NIN genes are activated by the NSP1–NSP2 complex in legumes, and NSP1 can directly bind to nodulation genes in M. trunctula [48] . Here, we show that GmNSP1s and GmNSP2s also positively regulate soybean nodulation, and GmNSP1a can activate GmNIN1a in soybean nodulation. Thus, NSP1/NSP2-mediated activation of NIN genes is a conserved mechanism that triggers the nodulation of legumes. Previously, we have shown that AON inhibits nodulation by suppressing the expression of GmNIN1a and the downstream genes [41] , but the underlying mechanism is still unknown. In this study, we used a protein–protein interaction approach to identify the GmRR11d as an interacting protein of GmNSP1a that negatively regulates nodulation. We proved that GmRR11d represses GmNIN1a expression through direct repression of GmNIN1a transcription and suppression of transcriptional activation activity of GmNSP1a on GmNIN1a expression. Our results showed that GmRR11d directly binds to the promoter of GmNIN1a to repress its transcription. In addition, GmRR11d through its C terminal can interact with the GRAS domain of GmNSP1a that is involved in its interaction with GmNSP2 and its DNA binding to suppress its transcriptional activity on GmNIN1a . Importantly, our data that increasing the protein quantity of GmRR11d decreases the ability of GmNSP1a to bind to the GmNIN1a promoter supports the hypothesis. Furthermore, we showed that repression of gene transcription by GmRR11d applies to all the GmNIN genes. Thus, GmRR11d can repress GmNINs expression by antagonizing the master upstream activator GmNSP1a to effectively inhibit nodulation. In addition to GmNSP1 and GmNSP2, CYCLOPS can also activate NIN expression during nodule formation [61] , [62] . It will be interesting to investigate whether GmRR11d interacts with and affects the transcriptional activity of CYCLOPS on the expression of GmNIN or other genes. Taken into account that GmRR11d is induced by CKs and its binding affinity to the promoter of GmNIN1a is enhanced by CKs, we proposed that AON may induce CK biosynthesis and GmRR11d to suppress NF signaling in inoculated roots. Since other GmRR11d paralog genes ( GmRR11a-c ) were differentially expressed during nodulation and these GmRR11s are highly conserved, we do not exclude the possibility that these genes also mediate nodulation inhibition by precise spatial-temporal modulation of CK response of infected root and nodulation activity. Type-B RR transcription factors, such as ARR10 in Arabidopsis , can regulate plant growth and development by targeting various genes in CK primary-response pathway and other regulatory signaling pathways [30] . Genome-wide identification of the target genes of GmRR11s will provide the molecular basis of transcriptional inhibition of nodulation and nodule development by AON and CKs. Legumes have evolved the AON systemic pathway to control the trade-off between plant growth and symbiotic nodulation [39] , [63] . It is conceivable that multiple mechanisms act to fine tune NF signaling and nodulation, but regardless of CK origin, the regulation of the CK level and CK sensitivity is central for optimal nodulation [26] , [30] , [33] . Based on our findings, we propose a model where AON induces GmRR11d through GmNARK during early root nodulation, which then inhibits further nodulation by simultaneously inducing CK hypersensitivity and repressing GmNIN expression and NF signaling (Fig. 7i ). At the early infection stage, GmNSP1s complexes with GmNSP2 to activate GmNIN expression when the level of GmRR11d is low and CK level is suitable for nodulation; while at the later stage of rhizobial infection, GmNSP1s binding to GmNIN promoters are effectively suppressed by increasing levels of GmRR11d and CKs at the onset of AON. In the meantime, high amount of GmRR11d can also directly bind to and repress the expression of GmNINs . The repression of GmNINs attenuates NF signaling activity after AON activation and blocks further rhizobial infection and nodule formation. Because NF, AON, CK biosynthesis and signaling are highly conserved in legumes [39] , [43] , [44] , [45] , [48] , our findings thus reveal the transcriptional regulation of NINs as a crucial interaction between CKs and NF/AON signaling pathways in the control of nodule number in legumes. Plant growth, hairy root transformation and rhizobium inoculation Soybean [ G. max (L.) Merrill cv. Williams 82, Bragg and the GmNARK mutant nts1007 in Bragg background] plants were used for gene cloning, gene expression and functional analysis of GmRR11d , GmNSP1/2 and GmNIN1a . Growth of soybean seedlings, hairy root transformation with Agrobacterium rhizogenesis strain K599 and inoculation with Bradyrhizobium ( B .) diaefficiens strain USDA110 were conducted as previously described [64] , [65] . Briefly, soybean seedlings were germinated and grown under 16 h/8 h light/dark conditions in a growth room at 25–26 °C.Young seedlings at 3–4 days after germination were used for hairy root transformation. For nodulation assays, transgenic composite plants were transplanted to pots containing vermiculite. The plants were grown for 1 week to allow rooting and then were inoculated with 30 mL B. diaefficiens strain USDA110 suspended in distilled water (OD 600 = 0.08). Nodule phenotypes were evaluated at 21 DAI or 28 DAI. DNA extraction and validation of transgenes Plant samples harvested from the composite plants were used for DNA extraction using the CTAB method as described previously [66] . Briefly, the hairy roots were ground in the isolation buffer (2% hexadecyltrimethylammonium bromide [CTAB], 1.4 M NaCl, 0.2% 2-mercaptoethanol, 20 mM EDTA, 100 mM Tris-HCl, pH8.0) and incubated at 60 °C for 30 min, DNA was then extracted with chloroform-isoamyl alcohol (24:1), after centrifugation (12000 × g for 10 min), the aqueous phase was transferred to clean tubes and the DNA was precipitated by ethanol. Presence of the Bar or Green fluorescent protein ( GFP ) gene was validated using PCR, and the hairy roots transformed with the corresponding empty vectors were used as negative controls. For the hairy roots harboring two genes, the presence of both Bar and GFP genes was detected by PCR. For confirming the edited hairy root in GmRR11d , GmNSP1a , GmNSP1b or GmNSP2a/b , the DNA fragments containing the sgRNAs were amplified and sequenced. 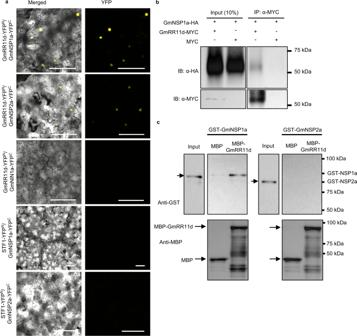Fig. 1: GmRR11d interacts preferentially with GmNSP1a. aBiFC assay to detect the interactions between GmRR11d and GmNSP1a or GmNSP2a. The interactions between GmRR11d and GmNIN1a41, GmNSP1a or GmNSP2a, and STF183were used as negative controls. Four independent experiments were repeated with similar results. Scale bars = 100 μm.bCoIP assay of interaction between GmRR11d and GmNSP1a. GmRR11d-6xMYC (58 kDa) alone or GmRR11d-6xMYC and GmNSP1a-3xHA (63 kDa) were transiently expressed under the control of the 35 S promoter inN. benthamianaleaves. GmRR11d-6xMYC immunoprecipitated from total protein extracts. Three independent experiments were repeated with similar results.cPull-down assays to show that MBP -GmRR11d (91 kDa) interacts with GST-GmNSP1a (87 kDa) but not GST-GmNSP2a (82 kDa). Three independent experiments were repeated with similar results. The primers for the Bar and GFP genes are listed in Supplementary Table 1 . RNA extraction and quantitative PCR analysis Total plant RNAs were extracted using TRIpure Reagent (Aidlab Biotechnologies Ltd., Beijing, China). Genomic DNAs were removed by gDNA Wiper Mix (Vazyme Biotech Co., Ltd., Nanjing, China). cDNAs were produced using a FastQuant RT Kit (Vazyme Biotech Co., Ltd.). qRT-PCR analyses were performed using SuperReal PreMix Plus (Vazyme Biotech Co., Ltd.). The primers used in qRT-PCR are listed in Supplementary Table 1 . Vectors construction For the proGmRR11d:GUS , 35 S : GmRR11d and RNAi-GmRR11d constructs, the promoter (2000 bp  upstream of ATG) or coding sequence of GmRR11d were amplified and cloned into pDONR207 by BP reactions. The resulting entry construct was inserted into pMDC162 ( proGmRR11d : GUS ), pEarlygate100-Flag ( 35 S : GmRR11d-Flag ) and pK7GWIWG2D(II) ( GmRR11d-RNAi ) through LR reactions. For the Cas9-GmRR11d , Cas9-GmNSP1a , Cas9-GmNSP1b and Cas9-GmNSP2a/b constructs, the sgRNAs were designed using CRISPR-P 2.0 software ( http://crispr.hzau.edu.cn/CRISPR2/ ) [67] . The pCBC-DT1T2 vector was used as the template to amplify the fragments with two sgRNAs, and then the fragments were connected to the skeleton vector pKSE401-GFP by Golden Gate reaction by the enzyme Bsa1 [68] , [69] . For the 35 S : GmNSP1a-GFP constructs, the coding sequence of GmNSP1a was amplified from cv. Williams 82 and inserted into pTF101-GFP vector using EcoRI and SalI . For subcellular localization, the coding sequences of GmRR11d , GmNSP1a , GmNSP2a were amplified and inserted into pTF101-GFP vector ( 35 S : GmRR11d-GFP ) or pEarlygate101-YFP vector ( 35 S : GmNSP1a-YFP and 35 S : GmNSP2a-YFP) . For the 35 S : GmRIC1 , 35 S : GmRIC2 and 35 S : GmTML1b constructs, the coding sequence of GmRIC1 , GmRIC2 and GmTML1b were amplified and cloned into pDONR207 by BP reactions. The resulting entry construct was inserted into pEarlygate100-Flag through LR reactions. Yeast two-hybrid assay To identify GmNSP1a-interacting proteins, we performed a Y2H screen using the Matchmaker GAL4 Yeast Two-Hybrid System (Clontech, USA), according to the manufacturer’s manual. RNA was extracted from mixture of roots and nodules using the RNeasy Plant Mini Kit (Qiagen) following the manufacturer’s instructions. Total RNA samples with an RNA integrity number >6.7 were used for the Y2H library construction. The cDNA library was constructed by OE Biotech (Shanghai, China). The full-length coding sequences of GmRR11d , GmNSP1a and GmNSP2a were amplified and the PCR products were cloned into the entry vector pDONR207 by BP reactions. pDONR207 harboring these genes were then ligated into pGBKT7 (BD) or pGADT7 (AD) by LR reactions. Yeast-two hybrid (Y2H) assays were done according to the Matchmaker GAL4 Two-Hybrid System (Clontech, Mountain View, CA). The β -Galactosidase activity of yeast cell was following the method of Möckli and Auerbach [70] . To further verify the interactions between GmRR11d/its domains and GmNSP1a/its domains, GmRR11d/GmNSP1a and their related domains were fused with the BD/AD domain in the pGBKT7/pGADT7 vector individually. For testing interactions, the above constructs were co-transformed into the yeast strain Saccharomyces cerevisiae AH109. Transformation was confirmed by growth on SD/-Leu/-Trp (SD/−2) medium. Interactions were assayed by spreading 2.5 μL of suspended transformed yeast on plates containing SD/-Ade/-His/-Leu/-Trp (SD/−4) medium. The interactions were observed after 3-4 days of incubation at 30 °C. The primers used in Y2H assays are listed in Supplementary Table 1 . BiFC assay The coding sequences of GmRR11d , GmNIN1a , STF1 , GmNSP1a and GmNSP2a were cloned into the pEARLYGAYE201-YN and pEARLYGAYE202-YC through the Gateway reaction system (Invitrogen, Carlsbad, CA), respectively. The constructs were transformed into Agrobacterium tumefaciens strain GV3101 for infiltration transformation of Nicotiana ( N .) benthamiana leaves. YFP fluorescence was detected using a Leica confocal laser scanning microscope (Leica Microsystems). For visualizing nuclei, leaves were stained with 2 mg/mL 4′, 6-diamidino-2-phenylindole (DAPI) for 10 min in dark conditions before observation. Localized surface plasmon resonance Protein-protein interactions were measured using an OpenSPR LSPR biosensor (Nicoya Life Science, Kitchener, Canada), as described previously [71] . In brief, 200 mL (50 μg/mL) of GST-GmRR11d was immobilized on a COOH sensor chip (Nicoya #SEN-AU-10012-COOH) at a flow rate of 20 mL/min in 1× PBS buffer (pH 7.4, RNase-free) and 0.1% (v/v) Tween 20. Free activated carboxyl groups were deactivated with the addition of 200 mL of blocking buffer (Nicoya). The immobilized protein was washed with running buffer (1× HEPES pH 7.4, 0.005% Tween 20) to reach a stable baseline. Buffer matched recombinant MBP-GmNSP1a (25 nM, 50 nM, 100 nM, 200 nM, 400 nM, 800 nM) or MBP-GmNSP2a (0.2 μM, 0.4 μM, 0.8 μM, 1.6 μM, 3.2 μM) was injected into the flow cell at a rate of 100 μL/min. Following a 5 min interaction time, the dissociation was recorded for an additional 7 min. Kinetic binding analysis was performed with the TraceDrawer software package (Ridgeview Instruments, Uppsala, Sweden). Sensorgram traces were fit to a 1:1 Langmuir model to derive affinity ( Kd ) constants. Pull-down assay The full-length coding sequence of GmRR11d was amplified and inserted into the pMAL-c2X vector (MBP-GmRR11d) (New England Biolabs). The full-length coding sequences of GmNSP1a and GmNSP2a were cloned into the pGEX-4T-1 vector (GST-GmNSP1a and GST-GmNSP2a) (GE Healthcare). The GmRR11d fused with MBP and GmNSP1a/GmNSP2a fused with glutathione S-transferase (GST) were expressed in Escherichia coli strain BL21 cells at 37 °C for 3 h and induced by 1 mM Isopropyl β-D-1-thiogalactopyranoside (IPTG). MBP-GmRR11d and GST-GmNSP1a/GmNSP2a were purified using amylose resin (New England Biolabs) or Pierce TM Glutathione Agarose (Thermo Fisher Scientific), respectively, according to the manufacturer’s instructions. Pull-down assays were performed as described previously [72] . The DNA-protein pull-down assay was performed as described by Vert et al. [73] , the biotinylated GmRR11d promoter was incubated with streptavidin MagBeads (GenScript, L00424) in TES buffer (10 mM Tris-HCl pH 7.5, 1 mM EDTA pH 8.0, 2 M NaCl) for 1 h at room temperature and then was washed three times in IP100 buffer (100 mM potassium glutamate, 50 mM Tris-HCl pH 7.6, 2 mM MgCl 2 , 0.05% v/v Nonidet P40). The MBP or MBP-GmRR11d was added to DNA-bound beads, and the mixture was rotated for 2 h at 4 °C. The beads were washed three times with IP100 buffer. The proteins were removed from the beads by boiling in 2× SDS loading buffer and subjected to PAGE. Co-IP assay The GmRR11d-MYC construct was co-expressed with GmNSP1a-HA construct in N. benthamiana leaves. Tobacco total proteins were extracted in extraction buffer (50 mM Tris-HCl, pH 7.5, 150 mM NaCl, 1 mM EDTA, 10% glycerol, 1% Triton X-100, 1 mM PMSF and 1× protease inhibitor cocktail and 10 μM ΜG132) and then were incubated with 8 µL anti-MYC agarose beads (SIGMA, A7470) for 2 h at 4 °C. The beads were washed five times with extraction buffer, and the immunoprecipitated proteins were eluted with SDS loading buffer with boiling for 5 min for western blotting. Samples were analyzed by western blot with anti-HA (SIGMA, SAB4300603, 1:2500) and anti-MYC (SIGMA, C3956, 1:2000). ChIP-qPCR assay Two grams of transgenic roots expressing 35 S : GmRR11d-FLAG , pEarlygate100-FLAG , 35 S : GmNSP1a-GFP , 35 S : GmRR11d - GmNSP1a-GFP and 35 S:GFP were used for ChIP assays. Roots were cross-linked with 1% formaldehyde at 4 °C for 10 min and neutralized with 0.125 M glycine. Roots were ground to fine power in liquid nitrogen and the nuclei isolated. Immunoprecipitation was done using anti-GFP (ab290, Abcam) or anti-FLAG (A2220, ANTI-FLAG M2 Affinity Gel, Sigma) antibodies. Chromatin precipitated without the use of antibodies was used as a negative control, while chromatin isolated before precipitation was used as an input control. qPCR analysis was performed, and soybean ELF1b ( GmELF1b ) was used as an internal control. The specific primers used in this experiment are listed in Supplementary Table 1 . Three independent biological repeats were performed for each analysis [41] . For the effect of exogenous cytokinin treatment on the binding activity of GmRR11d on the GmNIN1a promoter, two grams of transgenic roots (10 DAI) expressing EV1 and 35 S : GmRR11d-FLAG were treated with 0.1 μM 6-benzylaminopurine (BAP) for 4 h. The electrophoretic mobility shift assay The Electrophoretic Mobility Shift Assay (EMSA) was performed as described previously [41] . MBP, MBP-GmRR11d, GST, GST-GmRR11d, and GST-GmNSP1a proteins were expressed in E. coli cells and purified. EMSA assay was performed using Light Shift Chemiluminescent EMSA Kit (Pierce, Rockford, IL) according to the manufacturer’s protocol. The binding activity of the protein was analyzed using an oligonucleotide labeled with biotin at the 5′ end (Sangon Biotech). 200-fold unlabeled probe as a competitor were added to the reactions. For GmRR11d, the mutated probe sequence was changed from GGATT to AAAAA. The primers used in EMSA are listed in Supplementary Table 1 . Transcriptional repression of GmNIN1a by GmRR11d in plant cells A. tumefaciens strain GV3101 and A. rhizogenesis strain K599 were used for infiltration transformation of N. benthamiana leaves and hairy root transformation, respectively. The promoter of GmNIN1a was cloned into pCambia1391 vector to generate the reporter constructs proGmNIN1a : GUS (−2500 bp). The hairy roots expressing proGmNIN1a : GUS or proGmNIN1a-DM:GUS transformed with EV1 or 35 S : GmRR11d were inoculated with rhizobia for 3 days. For transiently co-expressing GmRR11d and GmNIN1a genes in N. benthamiana leaves, mixed culture with an equal volume (1:1) of each culture were used to inject the back of the leaves (the final OD 600 was 0.4 for each). At 48 h after injection, GUS expression was analyzed by GUS staining [61] . 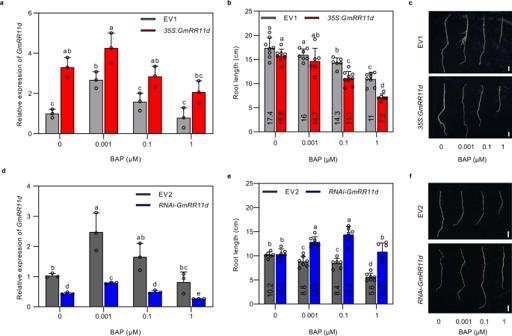Fig. 2: GmRR11d is CK responsive and positively regulates the sensitivity of soybean roots to CKs. aRelative expression ofGmRR11din transgenic roots expressing35S:GmRR11dtreated with BAP of different concentrations (0, 0.001, 0.1, 1 μM). The expression levels were normalized against the geometric mean of soybeanGmELF1b. Data are presented as means ± SD from three biological replicates. Different letters indicate significant differences atp< 0.05 (Two-way ANOVA).bLength of hairy roots expressing EV1 and35S:GmRR11dtreated with different concentrations (0, 0.001, 0.1, 1 μM) of BAP for 6 days (n≥ 6). Data are presented as means ± SE. Different letters indicate significant differences atp< 0.05 (Two-way ANOVA).cRepresentative images of individual root overexpressingGmRR11dand the EV1. Three independent experiments were repeated with similar results. Scale bars = 1 cm.dRelative expression ofGmRR11din transgenic roots expressingRNAi-GmRR11dtreated with BAP of different concentrations (0, 0.001, 0.1, 1 μM). The expression levels were normalized against the geometric mean of soybeanGmELF1b. Data are presented as means ± SD from three biological replicates. Different letters indicate significant differences atp< 0.05 (Two-way ANOVA).eLength of hairy roots expressing EV2 andRNAi-GmRR11dtreated with different concentrations (0, 0.001, 0.1, 1 μM) of BAP for 6 days (n≥ 6). Data are presented as means ± SE. Different letters indicate significant differences atp< 0.05 (Two-way ANOVA).fRepresentative images of individual root downregulatingGmRR11dand the EV2. Three independent experiments were repeated with similar results. Scale bars = 1 cm. DNA binding activity analysis of GmNSP1a to the promoter of GmNIN1a The constructs proGmNIN1a : GUS or proGmNIN1a-DM:GUS were transformed with EV1, 35 S : GmRR11d , 35 S : GmNSP1a and 35 S : GmRR11d + 35 S : GmNSP1a into N. benthamiana leaves. At 36 h after injection, GUS expression was analyzed by GUS staining. For β -glucuronidase (GUS) enzyme activity, N. benthamiana leaves were placed in a mortar containing liquid nitrogen, crushed, and then added with GUS enzyme extraction buffer (10 μL/mg tissue). The supernatant after centrifugation (12000 × g, 4 °C, 10 min) is the extract of GUS enzyme. The flourimetric assay of GUS activity were carried out by the methods, as described previously [74] . 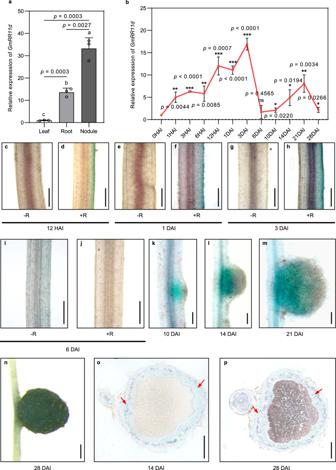Fig. 3: The expression pattern of GmRR11d during nodulation. a,bqRT-PCR analysis ofGmRR11dexpression in different tissues or during nodulation stages.aRoots, leaves, and nodules of soybean seedlings inoculated withB. diaefficiensstrain USDA110 were harvested at 28 DAI and used for gene expression analyses.GmELF1bwas used as the endogenous control gene. Data are presented as means ± SD from three biological replicates. More than 6 samples were analyzed in each independent biological repeat. Different letters indicate significant differences atp< 0.05 (One-way ANOVA).bSeven-day-old seedlings were inoculated withB. diaefficiensstrain USDA110 and the infected root materials were collected at 0, 1, 3, 6, 12 HAI and 1, 3, 6,10, 14, 21, 28 DAI for expression analysis ofGmRR11d.GmELF1bwas used as the endogenous control gene. The data are shown as the means ± SD from three biological replicates. Asterisks indicate significant differences relative to 0 HAI (Two-sided Student’st-test, *p< 0.05; **p< 0.01; ***p< 0.001).c–pHistochemical assay ofproGmRR11d:GUSand in the transgenic roots and nodules. Three independent experiments were repeated with similar results.c–jRepresentative GUS staining in hairy roots ofproGmRR11d:GUS. GUS activity was monitored at 12 HAIc,d, 1 DAIe,f, 3 DAIg,hand 6 DAIi,jwithB. diazoefficiensUSDA110. Scale bars = 100 μm inc–j.k–nThe expression pattern ofGmRR11din emerging nodulek, young noduleland mature nodulem,n.o,pCross-sectional analysis of the expression pattern ofGmRR11din young and mature nodules, the red arrows show cortex. Scale bars = 1 mm ink–p. In this experiment, protein concentrations were determined by using the Bradford’s dye binding assay [75] . 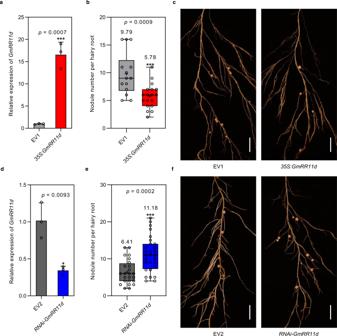Fig. 4: Alterations ofGmRR11dexpression affect nodulation. a–cOverexpression ofGmRR11dreduces nodule number.aqRT-PCR analysis of transgenic hairy roots expressing35S:GmRR11d. The expression levels were normalized against the geometric mean of soybeanGmELF1b. Data are presented as means ± SD from three biological replicates. Asterisks indicate significant differences relative to the EV1 control. Two-sided Student’st-test ***p0.001.b,cQuantification and representative images of nodule number per hairy root expressing EV1 and35S:GmRR11d. Data are presented as means ± SD (14 hairy roots in EV1 and 18 hairy roots in35S:GmRR11d). Three independent experiments were repeated with similar results. Asterisks indicate significant differences relative to the EV1 control. Two-sided Student’st-test, ***p< 0.001. Scale bars = 1 cm.d–fKnockdown ofGmRR11dincreases nodule number.dqRT-PCR analysis of transgenic hairy roots expressingRNAi-GmRR11d. The expression levels were normalized against the geometric mean of soybeanGmELF1b. Data are presented as means ± SD from three biological replicates. Asterisks indicate significant differences relative to the EV2 control. Two-sided Student’st-test, *p< 0.05.e,fNodulation phenotypic analysis of individual hairy roots expressing EV2 andRNAi-GmRR11dat 21 DAI. Scale bars = 1 cm. Data are presented as means ± SD (24 hairy roots in EV2 and 28 hairy roots inRNAi-GmRR11d). Three independent experiments were repeated with similar results. Asterisks indicate significant differences relative to the EV2 control. Two-sided Student’st-test, ***p< 0.001. Boxes indicate the first and third quartiles and the whiskers indicate the minimum and maximum values, the black lines within the boxes indicate the median values and black circles mark the individual measurements. The numbers above the boxes in (b) and (e) represent the mean values. Exogenous application of 6-benzylaminopurine For GmRR11d and GmRR15a/b expression in response to exogenous CK application, soybean seeds (W82) were germinated in vermiculite irrigated once with a low-nitrate solution. Seven-day-old seedlings were treated with 6-benzylaminopurine (BAP) using different concentrations for 3 h. PBS buffer was used as a control for analyzing the expression of GmRR11d and GmRR15a/b . To detect whether the expression of GmRR11d affects the sensitivity of soybean to cytokinin, empty vector (EV1) and 35 S:GmRR11d-FLAG vectors were used to hairy root transformation with A. rhizogenesis strain K599 using different concentrations (0, 0.001, 0.1, and 1 μM) of BAP. Grafting experiments The Bragg and nts1007 seeds used as scion and rootstock were seeded in vermiculite for germination (16 h light/8 h dark, 26 °C, 60% relative humidity). Ten-day-old seedlings were cut at the hypocotyl and grafted to reciprocal rootstock using 4 cm parafilm, then sealed with plastic film and cultured in dark condition for 3-4 days. It can be confirmed that the grafted seedlings survived when the first young trifoliate leaves show obvious signs of growth, then inoculated with B. diazoefficiens USDA110 and the shoots and roots were harvested at 4 days after inoculation. Histochemical analysis The infected hairy roots and nodules of soybean composite plants expressing proGmRR11d : GUS were stained with X-Gluc to test β -glucuronidase activity at the specified time points. Split-root assay The split-root experiments were carried out by the methods as described previously [76] . The seven-day-old Bragg and nts1007 roots were divided into two parts and treated with (+R) or without (-R) B. diazoefficiens strain USDA110. The roots (-R/-R, + R/-R, + R/ + R) were collected at 3 DAI and test the expression of GmRR11d . For the GUS staining of proGmRR11d:GUS in hairy root transformation system, the hairy roots were divided into two parts and treated with or without B. diazoefficiens strain USDA110. The hairy roots (-R/-R, + R/-R) were collected at 3 DAI. Phylogenetic analysis The protein sequences of G. max , M. truncatula and A. thaliana were obtained from Phytozome v12.1 database ( https://phytozome.jgi.doe.gov/ ) [77] and L. japonicus protein sequences were obtained from Miyakogusa.jp 3.0 database ( http://www.kazusa.or.jp/lotus/ ) and then imported into MEGA7.0 [78] for complete alignment using Explorer/Clustal [79] . The phylogenetic tree was built using MEGA7.0. Phylogenies were built using the neighbor-joining method with the bootstrapping value set at 1000 replications. Bioinformatics analysis The protein sequences were further characterized through a multiple sequence alignment via Clustal Omega hosted by EMBL-EBI ( https://www.ebi.ac.uk/Tools/msa/clustalo/ ). Synteny analysis was analyzed using TBtools software [80] . The gene structure analysis of GmNSP2a/b and the homologous genes were performed using GSDS 2.0 software [81] . 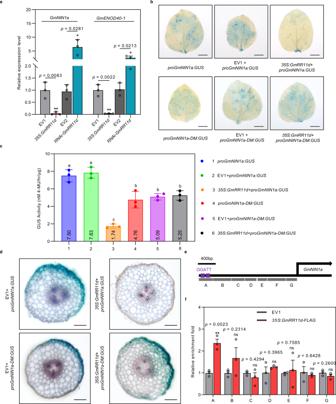Fig. 5: GmRR11d directly targets the promoter ofGmNIN1aand repressesGmNIN1aexpression. aqRT-PCR analysis ofGmNIN1aandGmENOD40-1expression in rhizobia-infected hairy roots expressing35S:GmRR11dorRNAi-GmRR11dat 2 DAI. The expression levels were normalized against the geometric mean of soybeanGmELF1b. Data are presented as means ± SD from three biological replicates. More than 12 roots were analyzed in three independent biological repeats. Asterisks indicate significant differences relative to the EV1 or EV2 control. Two-sided Student’st-test, *p< 0.05; **p< 0.005.b–dGUS assays showing the specific binding of GmRR11d to theGmNIN1apromoter and the inhibitory effect of GmRR11d onGmNIN1ainN. benthamianaleaf (b,c; Scale bars = 1 cm) and in transgenic soybean hairy root (d; Scale bars = 100 μm). TheproGmNIN1aandproGmNIN1a-DMcontain normal (GGATT) and mutated (AAAAA) GmRR11d binding sites inGmNIN1apromoter, respectively. The construct harboringproGmNIN1a:GUSorproGmNIN1a-DMwas co-transformed with empty vector (EV1) or35S:GmRR11dinto epidermal cells ofN. benthamianaleaves and transgenic hairy roots of soybean, and GUS staining were performed 48 h after transformation inN. benthamianaleaves and 2 DAI in transgenic hairy roots. Data are presented as means ± SD from three biological replicates. Different letters indicate significant differences atp< 0.05 (one-way ANOVA).eDiagram of theGmNIN1apromoters. GmRR11d binding site (GGATT) shown as purple boxes. The fragments marked by the letters A to G indicate the regions examined in ChIP-qPCR assays. Region A contains two GmRR11d binding sites.fChIP-qPCR assay showing binding of GmRR11d to theGmNIN1apromoter. DNA fragments were co-immunoprecipitated with anti-FLAG antibody from chromatin suspensions prepared from35S:GmRR11d-FLAGor empty vector (EV1) samples. DNA fragments corresponding to the regions indicated inewere analyzed by qRT-PCR. The DNA fragments were normalized to the input data. Data are presented as mean ± SD of three biological repeats. Asterisks indicate significant differences relative to the EV1 control. Two-sided Student’st-test, **p< 0.01. For protein alignment of ARR7 and ARR15 with their orthologs in soybean, protein sequences of GmRR15a/b/c/d, ARR7 and ARR15 were aligned using CLUSTALW website ( https://www.genome.jp/tools-bin/clustalw ) and visualized by ESPript 3.0 website ( http://espript.ibcp.fr/ESPript/cgi-bin/ESPript.cgi ) [82] . 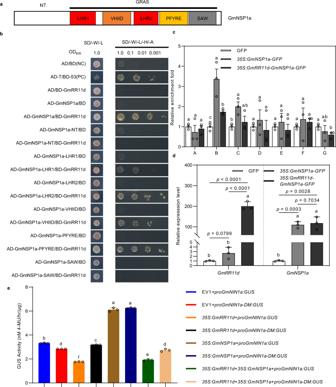Fig. 6: GmRR11d interacts with GmNSP1a and inhibits its transcriptional activity. aDomain structure of GmNSP1a.bDomain mapping for the interactions between GmNSP1a or its derivatives and GmRR11d by Y2H assay. Three independent experiments were performed with similar results.cChIP assay showing binding of GmNSP1a toGmNIN1apromoter and the inhibition effect of GmRR11d to the binding of GmNSP1a toGmNIN1apromoter. DNA fragments were co-immunoprecipitated with anti-GFP antibody from chromatin suspensions prepared from35S:GmNSP1a-GFP,35S:GmRR11d-GmNSP1a-GFPor control (empty vector) samples. DNA fragments corresponding to the regions indicated in Fig.5e. Data are presented as means ± SD of three biological repeats. Different letters indicate significant differences atP< 0.05 (One-way ANOVA).dThe expression level ofGmRR11dandGmNSP1ain hairy root expressing35S:GmNSP1a-GFPor35S:GmRR11d-GmNSP1a-GFP. Data are presented as means ± SD of three biological repeats. More than 30 hairy roots were analyzed in three independent biological repeats. Different letters indicate significant differences atP< 0.05 (One-way ANOVA).eGUS activity ofproGmNIN1a:GUSandproGmNIN1a-DM:GUSwith different combinations with35S:GmRR11d,35S:GmNSP1aand35S:GmRR11d+35S:GmNSP1ainN. benthamianaleaves. Data are presented as means ± SD from three biological repeats. Different letters indicate significant differences atP< 0.05 (One-way ANOVA). 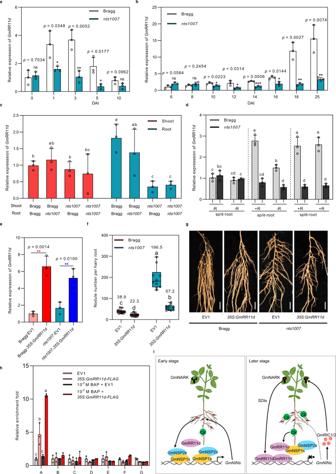Fig. 7: GmRR11d acts as a downstream regulator of GmNARK in soybean. a,bThe expression ofGmRR11din rootsaand nodulesbof wide-type cv Bragg andGmNARKmutantnts1007. Seven-day-old-plants were inoculated with USDA110. The roots were harvested at 0, 1, 3, 5, and 10 DAI and the nodules were harvested at 6, 8, 10, 12, 14, 16, 18, and 25 DAI. Data are presented as means ± SD from three biological repeats. More than 9 samples were analyzed in three independent biological repeats. Asterisks indicate significant differences relative to the wild type control. Two-sided Student’st-test, *p< 0.05;p** < 0.01; ***p< 0.001.cThe expression ofGmRR11din shoots and roots of Bragg/Bragg, Bragg/nts1007,nts1007/nts1007andnts1007/Bragg grafting plants. Data are presented as means ± SD from three biological repeats and 6 samples were collected for expression analysis. Different letters indicate significant differences atP< 0.05 (One-way ANOVA).dThe expression ofGmRR11din split-roots of Bragg andnts1007. -R/-R and +R/ + R treatment as negative and positive control. Data are presented as means ± SD from three biological repeats and 12 roots were collected for expression analysis. Different letters indicate significant differences atp< 0.05 (Two-way ANOVA)eqRT-PCR analysis ofGmRR11din empty vector (EV1) and35S:GmRR11dtransgenic hairy roots of Bragg andnts1007plants. Data are presented as means ± SD from three biological repeats and more than 10 roots were collected for expression analysis Asterisks indicate significant differences relative to the EV1 control. Two-sided Student’st-test, **p< 0.01.fNodule number of Bragg andnts1007plants expressing EV1 and35S:GmRR11dat 21 DAI. Data are presented as means ± SD from three biological repeats and more than 10hairy roots were collected for analysis. Different letters indicate significant differences atp< 0.05 (Two-way ANOVA).gPhenotypes of nodules from individual hairy roots of Bragg andnts1007plants expressing EV1 and35S:GmRR11dat 21 DAI.hBAP treatment increases the enrichment of GmRR11d in the promoter ofGmNIN1a. DNA fragments were co-immunoprecipitated with anti-FLAG antibodies from chromatin suspensions prepared from35S:GmRR11d-FLAGor control (EV1) samples treated with or without 10−7M BAP. The DNA fragments were normalized to the input data. Data are presented as means ± SD from three biological repeats. Different letters indicate significant differences atp< 0.05 (one-way ANOVA).iA proposed working model for GmRR11d-mediated nodulation inhibition. At low nitrogen conditions, rhizobia infection induces GmNSP1a to activateGmNIN1athat promotes nodulation and autoregulation of nodulation (AON). At the early infection stage, the level of GmRR11d is low and CK level is suitable for nodulation, GmNSP1s complexes with GmNSP2 to activateGmNINexpression; activation of AON induces expression of B-type regulator GmRR11d which interacts with GmNSP1a and suppresses its transcriptional activation ofGmNIN1a. Meanwhile, AON-induced CK accumulation enhances binding of GmRR11d to theGmNIN1apromoter to repress its expression induced by CK and to activate CK signaling, thereby inhibiting nodulation of soybean. Statistical analysis Data was analyzed using GraphPad Prism 8 (GraphPad Software, Inc., La Jolla, CA). Statistical significance was determined by ANOVA with Tukey’s post hoc test or the two-tailed Student’s t -test. The type of statistical significance test was described in the figure legends. Reporting summary Further information on research design is available in the Nature Portfolio Reporting Summary linked to this article.